Human cryptochrome exhibits light-dependent magnetosensitivity Humans are not believed to have a magnetic sense, even though many animals use the Earth's magnetic field for orientation and navigation. One model of magnetosensing in animals proposes that geomagnetic fields are perceived by light-sensitive chemical reactions involving the flavoprotein cryptochrome (CRY). Here we show using a transgenic approach that human CRY2, which is heavily expressed in the retina, can function as a magnetosensor in the magnetoreception system of Drosophila and that it does so in a light-dependent manner. The results show that human CRY2 has the molecular capability to function as a light-sensitive magnetosensor and reopen an area of sensory biology that is ready for further exploration in humans. In vertebrates, such as migratory birds and sea turtles, the ability to sense the Earth's magnetic field is clearly important for positional and directional information during their long-distance migrations [1] , [2] , [3] . In many animals, magnetoreception is thought to depend on light-sensitive chemical reactions involving the flavoprotein cryptochrome (CRY) [3] , [4] , [5] . There are two major groups of CRYs found in animals, based on both their phylogenetic position and function in the regulation of circadian clocks [6] . Drosophila -like type 1 CRYs (which have been found only in invertebrates) are sensitive to blue light and function mainly as circadian photoreceptors. On the other hand, vertebrate-like type 2 CRYs (which are found in both vertebrates and invertebrates) are thought to function mainly as negative regulators of the clockwork's transcriptional feedback loop and do so in a light-independent manner [7] . Genetic studies have shown that a light-dependent magnetic sense in Drosophila is indeed mediated by its type 1 CRY [8] , [9] . Furthermore, using the Drosophila GAL4-UAS transgenic approach for targeted gene expression, it has been shown recently that type 1 CRY proteins from either the fly itself or the monarch butterfly, and an insect version of type 2 CRY from the monarch can each restore magnetosensitivity and its light dependency in CRY-deficient Drosophila [10] . Humans are widely assumed not to have a magnetic sense [3] . For example, the extensive behavioural studies by Robin Baker [11] , [12] , [13] , [14] , [15] , suggesting a link between non-visual navigation and magnetoreception in humans, are controversial. However, there is consistent evidence of an influence of geomagnetic fields on the light sensitivity of the human visual system [16] , [17] . Moreover, it has been proposed recently that light-sensitive magnetic responses are not only used for directional information, but may also aid visual spatial perception in mammals, by providing a spherical coordinate system for integrating spatial position [3] . We therefore evaluated the light-dependent magnetosensing potential of human CRY. Here we show using a transgenic approach, that human CRY can function as a magnetosensor in the magnetoreception system of Drosophila and that it does so in a light-dependent manner. Thus, human CRY has the molecular capability to function as a light-sensitive magnetosensor, and this finding may lead to a renewed interest in human magnetoreception. Human CRY2 rescues light-dependent magnetosensitivity Although there are two versions of type 2 CRYs in humans (hCRY1 and hCRY2), we focused our transgenic study on hCRY2, because previous anatomical studies have shown that it is expressed at ca. 11-fold higher levels than hCRY1 in the retina [18] , [19] . Thus hCRY2 is nicely poised to receive the light information necessary to initiate a light-sensitive magnetic response in humans. In Drosophila , magnetosensitivity can be reliably examined using a behavioural assay, in which groups of individuals experience an electric-coil-generated magnetic-field gradient ranging from ambient to eight times the Earth's strength on one arm of a two arm T-maze [8] , [10] . The directional response of flies to the field is tested by comparing the number of flies in the arm that faces the coil that generates a magnetic field with the number in the opposite arm that faces the coil that is not magnetized. Flies are tested for their direction response in either the naive state or after training when the field is paired with a sucrose reward. Using this behavioural assay, both wild-type Canton-S flies and CRY-deficient flies expressing the Drosophila cry transgene under the control of the tim-GAL4 driver, which expresses the transgene where cry is normally expressed, manifest significant naive directional avoidance of the field (negative preference index value) and a significant directional trained preference for the field (positive preference index value) ( Fig. 1a , white and black bars, respectively) [8] , [10] . 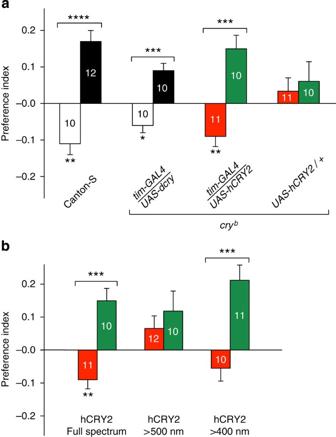Figure 1: Human CRY2 rescues light-dependent magnetoreception in CRY-deficient flies. (a) Atim-GAL4-driven humanCRY2transgene (tim-GAL4/UAS-hCRY2) rescues magnetic responses in the CRY loss-of-functioncrybmutant background. For comparison, naive and trained responses to the magnetic field are shown for wild-type Canton-S flies (left bar set; reproduced from ref.8) and for atim-GAL4-drivenDrosophila crytransgene incrybflies (tim-GAL4/UAS-dcry) (second from left bar set; reproduced from ref.10). TheUAS-hCRY/+transgene alone (without thetim-GAL4driver) did not result in significant magnetosentitive responses (P>0.05; right bar set). Bars show PI values for naive (white,dcry; or red,hCRY2) and trained (black,dcry; or green,hCRY2) groups. To test whether flies responded to the experimental magnetic field, we either used a one-samplet-test to compare naive PI values with zero (that is, PI value expected with no response to the magnetic field) or a Student'st-test to compare PI values between trained and naive groups. Numbers represent groups tested. Values are mean±s.e.m. *P<0.05; **P<0.01; ***P<0.001. Genotypes in parentheses:tim-GAL4/UAS-dcry(y w;tim-GAL4/UAS-mycdcry;cryb);tim-GAL4/UAS-hCRY(y w;tim-GAL4/UAS-mychCRY2;cryb); andUAS-dcry/+(y w;UAS-mychCRY2/+;cryb). (b) Light dependence of magnetic responses rescued by human (h)CRY2 (y w;tim-GAL4/UAS-mychCRY2;cryb). The full-spectrum data are the same as those depicted ina. The irradiance curves for the three light conditions used are the same as those used previously8. Bars show PI values for naive (red) and trained (green) groups. To test whether flies responded to the experimental magnetic field, we either used a one-samplet-test to compare naive PI values to zero (that is, PI value expected with no response to the magnetic field) or a Student'st-test to compare PI values between trained and naive groups. Numbers represent groups tested. Values are mean±s.e.m. **P<0.01, ***P<0.001. Figure 1: Human CRY2 rescues light-dependent magnetoreception in CRY-deficient flies. ( a ) A tim-GAL4 -driven human CRY2 transgene ( tim-GAL4/UAS-hCRY2 ) rescues magnetic responses in the CRY loss-of-function cry b mutant background. For comparison, naive and trained responses to the magnetic field are shown for wild-type Canton-S flies (left bar set; reproduced from ref. 8 ) and for a tim-GAL4 -driven Drosophila cry transgene in cry b flies ( tim-GAL4/UAS-dcry ) (second from left bar set; reproduced from ref. 10 ). The UAS-hCRY/+ transgene alone (without the tim-GAL4 driver) did not result in significant magnetosentitive responses ( P >0.05; right bar set). Bars show PI values for naive (white, dcry ; or red, hCRY2 ) and trained (black, dcry ; or green, hCRY2 ) groups. To test whether flies responded to the experimental magnetic field, we either used a one-sample t -test to compare naive PI values with zero (that is, PI value expected with no response to the magnetic field) or a Student's t -test to compare PI values between trained and naive groups. Numbers represent groups tested. Values are mean±s.e.m. * P <0.05; ** P <0.01; *** P <0.001. Genotypes in parentheses: tim-GAL4/UAS-dcry ( y w ; tim-GAL4/UAS-mycdcry ; cry b ); tim-GAL4/UAS-hCRY ( y w ; tim-GAL4/UAS-mychCRY2 ; cry b ); and UAS-dcry/+ ( y w ; UAS-mychCRY2/+ ; cry b ). ( b ) Light dependence of magnetic responses rescued by human (h)CRY2 ( y w ; tim-GAL4/UAS-mychCRY2 ; cry b ). The full-spectrum data are the same as those depicted in a . The irradiance curves for the three light conditions used are the same as those used previously [8] . Bars show PI values for naive (red) and trained (green) groups. To test whether flies responded to the experimental magnetic field, we either used a one-sample t -test to compare naive PI values to zero (that is, PI value expected with no response to the magnetic field) or a Student's t -test to compare PI values between trained and naive groups. Numbers represent groups tested. Values are mean±s.e.m. ** P <0.01, *** P <0.001. Full size image Remarkably, CRY-deficient flies expressing the hCRY2 transgene under the control of the tim-GAL4 driver also showed comparably robust naive and trained responses to a magnetic field under full-spectrum light ( Fig. 1a , red and green bars, respectively), while CRY-deficient fly lines expressing either the GAL4 driver alone [10] or the UAS-hCRY2/+ transgene alone ( Fig. 1a ) did not respond. Moreover, the hCRY2 rescue of magnetosensitivity was light sensitive ( Fig. 1b ); the hCRY2-induced magnetic responses were blocked when only long-wavelength light (>500 nm) was available, and were partially restored when light >400 nm was available. Thus, light in the blue range is necessary for the hCRY2 magnetic response. Our results show that hCRY2, the prototype type 2 CRY [18] , [19] , has the molecular capability to function in a light-dependent magnetoreception system, either as a light-sensitive magnetosensor or as part of a magnetosensing pathway. However, we do not yet know whether this capability is translated into a downstream biological response in the human retina. Nonetheless, the transgenic findings with hCRY2, together with its anatomical location in the human retina and previous work showing field effects on the visual system, suggest that a reassessment of human magnetosensivitiy may be in order. The results also define a clear light-sensitive response for a mammalian CRY, as predicted in 1998 (ref. 18 ). Additional research on magnetosensitivity in humans at the behavioural level, with particular emphasis on the influence of magnetic fields on visual function, rather than non-visual navigation, would be informative. Fly lines Fly stocks were raised on standard cornmeal/agar medium at 25 °C and 60% relative humidity under a 12-h light:12-h dark lighting cycle. The cry b and UAS-dcry ( UAS-mycdcry ) were a gift from Patrick Emery. The tim-GAL4 ( tim-GAL4/CyO ) [20] driver line was used for transgene expression in cry b flies. For generating UAS–mychCRY2 transgenic lines, the hCRY2 open reading frame was amplified by PCR from pfmh2 and subcloned into the Bgl II and Not I sites of the pUAST attBmyc vector. The myc-pUASTattB vector was generated by cloning a Bam HI-myc- Bgl II fragment, created using two oligos followed by primer extension, into the Bgl II site of pUASTattB. The construct contained a full Kozak sequence. The construct was sequenced before injection into y w , nos-phiC31/+ ; attP40 or y w , nos-phiC31/Y ; attP40/+ embryos by Genetic Services. During balancing, the y w , nos-phiC31 -containing X chromosome was replaced with the y w -containing X chromosome. Behavioural apparatus The apparatus consisted of a choice chamber and an illuminated black box containing the two-coil system connected to an adjustable DC power supply [8] . The choice chamber was comprised of a one-tube training section and a two-tube choice section (T-maze) for testing the relative response of flies to a magnetic field. An elevator section was used to transfer flies between training and T-maze sections (see below). The housing box was constructed such that the choice chamber could be placed between the two coils in either an upright position (used during training) or when rotated to the horizontal (used during testing). In this way, flies were exposed to the same lighting conditions and magnetic field intensity during training and test trials. The two-coil system allowed for the production of a magnetic field on one side, while producing no field on the opposite side and alternation of the field between sides; heat was generated equally in either coil, with or without generating a magnetic field. Coils were positioned directly under the tube ends at 45° to the horizontal. We adjusted the power supply so that the magnetic field intensity ranged from 0.1 G at the tube entrance to 5 G at the end of the tube. The box containing the coil system was open on the top so that the chamber, regardless of position, could be illuminated by one ZooMed Reptisun 10.0 UVB fluorescent tube (F17T8). Irradiance measurements were taken from inside one arm of the T-maze portion of the choice chamber apparatus to ensure that the lighting conditions measured represented those experienced by the flies while they were being either trained or tested. Wavelength dependence of magnetosensitivity was examined by either covering the top of the box with a long-wavelength filter that transmitted wavelengths of light >500 nm (Edmund Optic) or >400 nm (E400 from Gentex). Behavioural procedure Flies were starved for 18 h before testing their magnetic response. All experiments were performed between 0800 and 1500 hours EST. Flies in the trained group were moved into the training section facing one of two adjustable coils with no field for 2 min, and then were reloaded into the training tube containing sucrose reinforcement and a magnetic field for an additional 2 min. After being held for 1 min in the elevator section, flies were tested for their magnetic preference by transferring them to the T-maze section and allowing them to choose between the sides with or without a magnetic field for 2 min. Flies in the naivegroup were loaded into the elevator section and immediately transferred to the T-maze and allowed to choose between the sides with or without a magnetic field for 2 min. Trained and naive groups were tested consecutively with the magnetic field on the same side. As an additional control for side preferences independent of magnetic stimuli, we tested flies in the absence of a magnetic field. For each population of flies tested (100–150 individuals), we calculated a preference index (PI) value based on the following equation: (P M -0.5)/0.5, where P M is the proportion of flies on the magnetic field side of the T-maze. To test whether flies responded to the experimental magnetic field, we either used a one-sample t -test to compare naive PI values to zero (that is, PI value expected with no response to the magnetic field) or a Student's t -test to compare PI values between trained and naive groups. How to cite this article: Foley, L. E. et al . Human cryptochrome exhibits light-dependent magnetosensitivity. Nat. Commun. 2:356 doi: 10.1038/ncomms1364 (2011).